Hydrochromic molecular switches for water-jet rewritable paper The days of rewritable paper are coming, printers of the future will use water-jet paper. Although several kinds of rewritable paper have been reported, practical usage of them is rare. Herein, a new rewritable paper for ink-free printing is proposed and demonstrated successfully by using water as the sole trigger to switch hydrochromic dyes on solid media. Water-jet prints with various colours are achieved with a commercial desktop printer based on these hydrochromic rewritable papers. The prints can be erased and rewritten dozens of times with no significant loss in colour quality. This rewritable paper is promising in that it can serve an eco-friendly information display to meet the increasing global needs for environmental protection. Although we live in an age dominated by electronic displays, paper prints still play a crucial role in our daily lives. Even though the initial cost of office printing setup is relatively low, actual cost of its on-going usage can be quite substantial because of frequent replacement of expensive ink cartridges. In addition, several international surveys reported that 90% of all information in businesses is currently retained on paper, and most of the prints are only used for one-time reading before being disposed [1] . Current digital prints do not de-ink and recycle well, and this creates huge problems of solid waste and environmental pollution. Ink-free printing and rewritable paper [2] , [3] , [4] , [5] , [6] , [7] , [8] , [9] , [10] have recently attracted attention owing to their potential benefits to forest conservation [11] , waste paper reduction and cutting down the cost of office printing. Incorporating switchable dyes in paper as an imaging layer represents an ideal economic approach towards rewritable paper. Leuco dyes [12] , [13] and photochromic compounds [14] , [15] have attracted much attention as new rewritable imaging dyes for rewritable paper. In particular, spiropyrans and related molecular switches, which are well known to undergo light-stimulated reversible isomerizations [16] , [17] , [18] , [19] between ring-closed forms (CFs) and ring-open forms (OFs) accompanied by significant colour changes, might be suitable candidates for the development of rewritable paper [20] , [21] . However, the prevailing colour-switching stimuli for these molecules are mainly UV/Vis [22] , [23] and acid/base [24] , [25] , which lead to problems, such as molecular degradation, potential safety issues and environmental hazards. These problems limit greatly their practical applications. From a green perspective [26] , it would be ideal if water can be used as the trigger to stimulate molecular switches for the development of rewritable paper. As water is a renewable resource and obviously poses no risk to the environment, its introduction and removal can be safely achieved, and water integrates well with fully developed ink-jet printing techniques (here for convenience, the water-triggered switchable dyes are named hydrochromic dyes, and printing with water only instead of ink is called water-jet printing). However, little progress has been made in this respect because of some major challenges. Specifically, the dye molecule should (i) exist in only one of its two states in the absence or presence of water, respectively, with high preference, (ii) be capable of integration into paper-based materials, where the hydrochromic behaviour still lives on and (iii) the resulting paper materials should be stable and robust enough to endure many write and erase cycles under ambient or mild conditions. Herein, we systemically screen three types of 18 structurally related switchable molecules in order to investigate the structure–hydrochromic property relationship in solution and evaluate their potential as water-triggered imaging materials. We then investigate the performances of candidate dyes in the solid state. Finally, we develop a prototype of rewritable paper using suitable hydrochromic dyes, which integrates well with current ink-jet printing techniques and demonstrates the reversibility and stability, indicating the promising real application of these materials. Screening for suitable hydrochromic dyes Inspired by the literature [27] , [28] , [29] , [30] , [31] studying solvation effects on the isomerization of some spiropyrans in aqueous solutions, we conjectured that the spiropyrans and related molecular switches could be potential hydrochromic dyes. By reviewing existing solvatochromic results of spiropyrans and related molecular switches reported so far, one critical problem preventing them being used practically is the colour instability under ambient light [27] , [28] , [29] . This might be due to unfavourable conjugated push–pull zwitterionic structure of their merocyanine isomers, which readily undergoes the ring-closing reaction under visible light. We assumed that breaking the conjugated linkage of the zwitterions could improve their colour stability. In order to prove our assumption, we have designed and synthesized three classes of 18 structurally related switchable molecules—oxazolidines ( 1 – 10 ), oxazines ( 11 – 13 ) and spiropyrans ( 14 – 18 ) ( Fig. 1a ). 1 – 10 were synthesized [19] , [32] with a modified four-step procedure by using phenylhydrazines as starting materials, as shown in Fig. 2 . First, 2,3,3-trimethylindolenine intermediates were obtained by the classical method of Fischer indole synthesis. These indolenines are then quaternized with 2-bromoethanol to afford indoleninium bromides, which are subsequently treated with the corresponding aromatic aldehydes in ethanol with CH 3 SO 3 H as a catalyst to obtain precipitated condensation products. At last, the CFs of 1 – 10 were obtained by basic treatment of condensation products with 5% NaHCO 3 aqueous solutions and extraction with ethyl acetate. 11 – 13 were synthesized [33] , [34] according to the work reported by F. M. Raymo’s group and us. 14 – 18 were synthesized and purified according to literature [27] , [35] , [36] . The detailed synthesis and characterization information for 1 – 18 was supplied in Supplementary Methods . 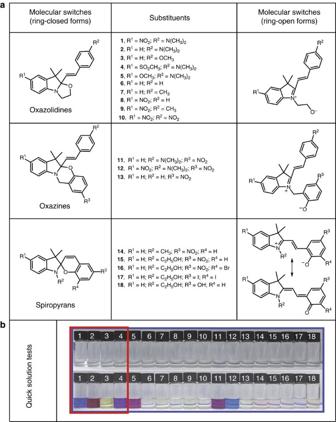Figure 1: Molecule design and screening for suitable hydrochromic dyes. (a) Structures of the investigated three classes of molecular switches1–18in their ring-closed forms and ring-open forms with different substituents and (b) the results of their quick solution tests (Photographs of solutions of1–18in 1,4-dioxane (2 ml,C=1 × 10−4mol l−1) before (above) and after (below) adding 2 ml of water at ambient conditions. The suitable hydrochromic dyes are marked by red frame. Figure 1: Molecule design and screening for suitable hydrochromic dyes. ( a ) Structures of the investigated three classes of molecular switches 1 – 18 in their ring-closed forms and ring-open forms with different substituents and ( b ) the results of their quick solution tests (Photographs of solutions of 1 – 18 in 1,4-dioxane (2 ml, C =1 × 10 −4 mol l −1 ) before (above) and after (below) adding 2 ml of water at ambient conditions. The suitable hydrochromic dyes are marked by red frame. 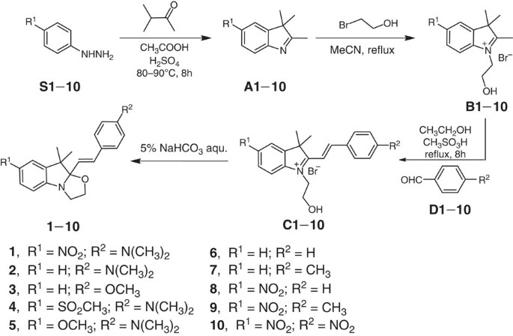Figure 2: General route for synthesis of1–10. Preparation of oxazolidines1–10starts with various substituted phenylhydrazines (S1–10); they are converted to corresponding 2,3,3-trimethylindolenine (A1–10) first, indoleninium bromides (B1–10) next, condensation intermediates (C1–10) then and finally to the desired target molecules (1–10). ‘aqu.’ is the abbreviation for aqueous solution. Full size image Figure 2: General route for synthesis of 1–10 . Preparation of oxazolidines 1 – 10 starts with various substituted phenylhydrazines ( S1 – 10 ); they are converted to corresponding 2,3,3-trimethylindolenine ( A1 – 10 ) first, indoleninium bromides ( B1 – 10 ) next, condensation intermediates ( C1 – 10 ) then and finally to the desired target molecules ( 1–10 ). ‘aqu.’ is the abbreviation for aqueous solution. Full size image Quick solution tests of the hydrochromic properties of 1 – 18 were conducted first in 1,4-dioxane/water binary solvent systems ( Fig. 1b ). To our pleasant surprise, most of oxazolidines ( 1 – 5 ) and oxazines ( 11 – 12 ) have favourable hydrochromic properties with good colour intensity and stability at ambient conditions, while the well-studied conventional spiropyrans ( 14 – 18 ) hardly show hydrochromism under the same conditions, and their OFs can only be observed either at elevated temperature or in the dark with poor colour intensity (more than one order of magnitude lower) (see Supplementary Fig. 1 and Supplementary Discussion ). Furthermore, oxazolidines or oxazines can be converted exclusively to their coloured OFs with water at room temperature (see Supplementary Fig. 2 ). Conjugated substituents conjoined to molecular structures usually play important roles on their properties, such as sensitivity, solubility, molecular colour and colour intensity. To verify how various substituents actually affect these properties of our molecules, a dual-correlation screening of both wavelength and intensity of the maximum absorption peak against the water content is used (see Supplementary Fig. 1 ). The results show that 5 and 11 are very labile to ambient polarity, and 12 has poor solubility in aqueous solution. It needs to be mentioned that a non-conjugated functional effect on molecular colour has also been discovered herein—that is, the wavelength of the maximum absorption peak red shifts in the case of 11 versus 2 or 12 versus 1 (nitrophenoxide versus ethoxide substitute on nitrogen), which have the same positively charged colour-dominating backbones in their OFs (see Supplementary Fig. 1b and Supplementary Discussion ). The screening results indicate that oxazolidines with electron-donating groups on R 2 and either electron-withdrawing groups on R 1 or none, such as 1 – 4 , are good candidates for hydrochromic dyes because of their desired properties of good solubility, fast switchability, fine-tunable chroma, excellent colour intensity and stability. Reversible hydrochromic behaviour of 1 We take 1 as an example herein to show clearly in detail the reversible hydrochromic behaviour between its ring-closed isomer 1 C and ring-open isomer 1 O in EtOH-H 2 O solutions ( Fig. 3a ). Without water, only one broad hump absorption band can be observed at wavelengths <440 nm, which indicates that 1 exists completely as 1 C in ethanol. Upon increasing the water content ( Fig. 3b ), a new absorption band centred at 588 nm (presumably 1 O ) is observed with an isosbestic point at 440 nm and increases along with a gradual decrease of its original hump absorption. 1 H NMR spectroscopy of this hydrochromic reaction also firmly supports the changes from 1 C to 1 O (see Supplementary Fig. 3 ). As the water content is decreased (see Supplementary Fig. 4 ), the absorption band associated with the 1 O at 588 nm gradually diminishes with the same isosbestic point. The microenvironment with multi-molecular hydrogen-bonding networks [27] , [28] plays an important role for this water-induced switching phenomenon from 1 C to 1 O , which was demonstrated by the fact that an equilibrium of both 1 C and 1 O coexsits also in some other protic solvents—that is, methanol and ethylene glycol (see Supplementary Fig. 5 , Supplementary Table 1 and Supplementary Discussion ). Water with both properties of a larger dipole and better hydrogen-bond donator can significantly reduce the energy of 1 O more than 1 C . The energy of 1 O becomes lower than 1 C when the water content reaches a certain amount enough, to support a better solvato-microenvironment, consequently shifting equilibrium from 1 C to 1 O (see Supplementary Fig. 6 ). These results indicate that the water-triggered molecular switching process is in thermodynamic control. The equilibrium constant K eq =0.113 for 1 in CD 3 OD/H 2 O has been calculated based on 1 H NMR data (see Supplementary Fig. 7 and Supplementary Note 1 ). The observation of this fully reversible hydrochromic property of 1 demonstrates its potential application as a water-triggered imaging material. 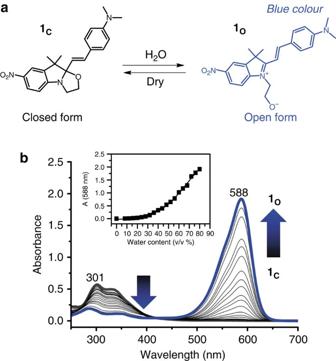Figure 3: Water-triggered reversible isomerization of1in solution. (a) The illustration of reversible water-stimulated isomerization between ring-closed and ring-open isomers for1. (b) UV–vis absorption spectra of1in variable mixtures of ethanol and water with increasing percentage of water by volume from 0 to 80% (C=2 × 10−5mol l−1, 20 °C, seeSupplementary Methods). Inset: Plot of absorbance atλmax=588 nm with water content. Figure 3: Water-triggered reversible isomerization of 1 in solution. ( a ) The illustration of reversible water-stimulated isomerization between ring-closed and ring-open isomers for 1 . ( b ) UV–vis absorption spectra of 1 in variable mixtures of ethanol and water with increasing percentage of water by volume from 0 to 80% ( C =2 × 10 −5 mol l −1 , 20 °C, see Supplementary Methods ). Inset: Plot of absorbance at λ max =588 nm with water content. Full size image Structure design of the water-jet rewritable paper An ethanol solution of 1 C was then directly soaked into a paper substrate to further investigate whether its reversible hydrochromic behaviour still lives on in the solid state. Unfortunately, to our surprise, a stable blue colour of 1 remains on the paper after solvent evaporation even in the absence of water. The same phenomenon is observed also with other polyhydroxyl substrates, such as silica gel, and polyvinyl alcohol, but does not appear on non-hydroxyl substrates, such as glass, non-cellulose filter paper, polyester and nylon. These results indicate that microenvironments play a crucial role to stabilize thermodynamically certain isomers, and the stable blue colour of 1 is closely related with the polyhydroxyl microenvironment, which favours the 1 O thermodynamically. This conclusion is further supported by the experimental observation that the blue colour can be switched to colourless with base and returned back to blue with acid (see Supplementary Fig. 8 ). By analysing the difference between ethanol solution and the solid substrates, we hypothesize that the undesired conversion of 1 C to 1 O is caused by the presence of an immobile polyhydroxyl microenvironment and stable spatial multi-hydroxyl participation, which might provide much better stabilization to 1 O than the mobile multi-hydroxyl environment in ethanol. This phenomenon observed herein is conceptually similar to some cases of reactions that proceed easily in an immobile microenvironment of an enzyme but do not happen in solution. We assume that passivation of the hydrogen bonding of the polyhydroxyls of paper might be a key to solve the problem. Consistent with this hypothesis are the facts that the stable blue colour of 1 on paper can be reconverted back to colourless by post-treatment with dimethyl sulfoxide (DMSO), a hydrogen bond acceptor, and the colour of this revived 1 on the cellulose paper can be reversibly switched back with water. In addition, the unwished blue colour of 1 O can also be avoided when the paper substrate is pretreated with DMSO before loading 1 C . For practical application, non-volatile polyethylene glycol (PEG) as a hydrogen bond acceptor proved to be a better material than DMSO for modification of the paper cellulose. Other challenges preventing the dye from being used practically in the solid state were also encountered and successfully overcome, such as unwanted colouration in damp air, long colour developing time because of slow water penetration, quick fading of the colour because of fast water evaporation under relatively warm and dry conditions, and the formation of microcrystalline aggregates of 1 C . Microcrystalline aggregates are not switchable, which is supported by the observation that the khaki powder of 1 C does not undergo colour change after its exposure to water. To solve these problems, a prototype of a four-layer structure to be employed as rewritable paper, abbreviated as RP , has been developed with the help of PEG to enhance its practical usability against various extreme real life situations. PEG not only passivates efficiently the hydroxyl groups of paper but also possesses excellent swellability for water, which facilitates the penetration of water molecules, and consequently increases the opportunity of triggering the ring-opening isomerization of 1 C . In addition, PEG also acts as a solid state solvent and prevents 1 C from forming the non-switchable microcrystalline aggregates. Incorporating hydrating additives is usually effective in extending the lasting time of water prints. To improve the legible colour-lasting time, various hygroscopic salts (that is, NaCl, CaCl 2 , NaNO 3 , CH 3 COONa and CH 3 COONH 4 ) have been investigated for the RP , and NaNO 3 was the one selected in our system. The four layers of the RP structure ( Fig. 4a ) include: (i) the bottom layer consisting of the paper substrate, (ii) a passivation layer consisting of PEG directly in contact with the paper substrate as a means to prevent hydrogen bonding between 1 C and the exposed donors on the paper surface, (iii) a thin film of PEG in which 1 C is ‘dissolved’ serving as the imaging layer along with NaNO 3 as the hydrating additive to extend the image lifetime and (iv) a final layer of PEG coated on the surface acting as an overcoat to prevent not only the undesired colouration caused by a damp atmosphere but also problems of any possible dye leakage and potential dye exposure upon human contact. We have successfully printed on the paper by water-jet printing using a commercially available ink-jet printer with a cartridge filled purely with water ( Fig. 4b ). At present, the minimum amount of water for the colour appearance of the prints in our water-jet printing system is found to be 12 pl per colour dot based on HP deskjet 2010 printer (see Supplementary Fig. 9 ). Good resolution of the blue prints in size 10.5 has been achieved so far with current water-jet printing, and the legibility of the prints can last 22 h under ambient condition (T<35 °C, humidity 20–80%), which is long enough for the purposes of temporary reading. The rate of the colour developing with water is found to be in less than 1 s, and this means that the colour appears instantly during the water-jet printing from a practical perspective. The prints can also be erased quickly by mild heating. The rates of colour disappearance varied with the heating temperature, and it takes about 30 s to vanish the colour prints at 70 °C. Dedicated efforts are being given to further improve both resolution and image-lasting time. 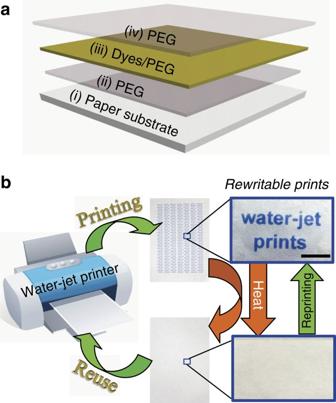Figure 4: Structural design and water-jet printing of RP. (a) Schematic illustrations of the four-layer structure used to create theRPmaterials based on1. (i) Filter paper is used as the substrate layer; (ii) PEG is used as the passivation layer; (iii) a thin film of PEG in which1Cis dissolved serves as the imaging layer; (iv) a film of PEG coated on top acts as a protection layer. (b) Schematic illustrations of a printing-reuse cycle of paper based on water-jetRP. Photographs of the letters produced by water-jet printing on thisRP(above) followed erasing of those images by mild heating (below). Scale bar=5 mm. Figure 4: Structural design and water-jet printing of RP. ( a ) Schematic illustrations of the four-layer structure used to create the RP materials based on 1 . (i) Filter paper is used as the substrate layer; (ii) PEG is used as the passivation layer; (iii) a thin film of PEG in which 1 C is dissolved serves as the imaging layer; (iv) a film of PEG coated on top acts as a protection layer. ( b ) Schematic illustrations of a printing-reuse cycle of paper based on water-jet RP . Photographs of the letters produced by water-jet printing on this RP (above) followed erasing of those images by mild heating (below). Scale bar=5 mm. Full size image Reversibility and colour variety of the rewritable prints Reflective UV–vis spectroscopy was used to test the reversibility and repeatability. In the absence of water, the RP material exhibits a hump absorption band centred around 301 nm, which is the characteristic feature of 1 C . Upon introduction of water, a new absorption band centred at 592 nm associated with 1 O is observed, accompanied by the diminishment of the one centred at 301 nm ( Fig. 5a ). The reflectivity at 592 nm was recorded after repetitive writing with water spraying and erasing by heating at 70 °C. It is found that only a slight decrease in colour intensity is observed after more than 10 consecutive write–erase cycles ( Fig. 5b ), and no colour can be detected from the back side of the paper after dozens of rewritings. This indicates that the reversible hydrochromic switching behaviour of 1 can be retained in the RP material, and 1 can be immobilized in the imaging layer without leaking. 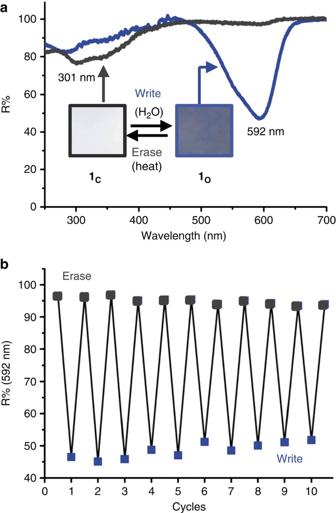Figure 5: Reversibility and repeatability of hydrochromic RP. (a) The reflective UV-vis spectra of theRPintegrated with1before (black trace) and after (blue trace) addition of water, at which points the material turns from a white to a dark blue, respectively. The size of the photographs for rewritable papers is 40 mm by 40 mm. (b) A plot of the reflectivity at 592 nm versus the number of cycles as theRPmaterial is cycled through water spraying (write) and water removal (erase) by means of heating at 70 °C. Figure 5: Reversibility and repeatability of hydrochromic RP. ( a ) The reflective UV-vis spectra of the RP integrated with 1 before (black trace) and after (blue trace) addition of water, at which points the material turns from a white to a dark blue, respectively. The size of the photographs for rewritable papers is 40 mm by 40 mm. ( b ) A plot of the reflectivity at 592 nm versus the number of cycles as the RP material is cycled through water spraying (write) and water removal (erase) by means of heating at 70 °C. Full size image Different colours of RP can also be achieved using suitable hydrochromic dyes. For example, the oxazolidines 2 , 3 and 4 can also be reversibly switched to their CFs by water, which exhibit magenta, gold and purple colours when stimulated with water, respectively (see Supplementary Fig. 10 ). After integration of these dyes using similar procedures to 1 on the paper substrate, RP s showing magenta, gold and purple characters can be obtained by water-jet printing ( Fig. 6 ). At present, our rewritable papers are in the monochromic stage of development. Multicolour rewritable paper with longer image lifetime is currently under investigation. 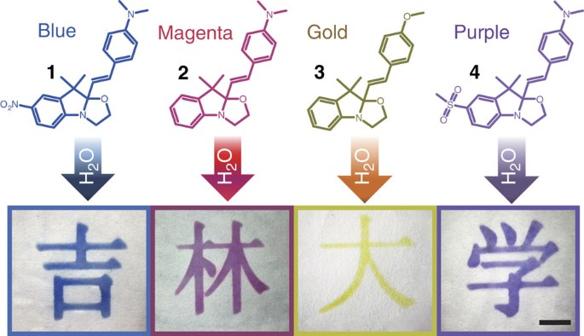Figure 6: Water-jet prints with different colours. Different colours ofRPscan be achieved by integration of1–4, respectively. The four Chinese characters shown, which mean Jilin University, were printed by water-jetting. Scale bar=1 cm. Figure 6: Water-jet prints with different colours. Different colours of RPs can be achieved by integration of 1 – 4 , respectively. The four Chinese characters shown, which mean Jilin University, were printed by water-jetting. Scale bar=1 cm. Full size image On the basis of the knowledge on relationship of the molecular structures to their hydrorchromic properties obtained from this study, we can anticipate that halochromic oxazines with appropriate functional groups pioneered by Professor F.M. Raymo’s group [37] , [38] , [39] may also be used as hydrochromic materials. As regards to toxicity and safety issues of the rewritable materials in specific and extreme exposure situations, the cytotoxicity tests of 1 – 4 have been conducted in HeLa cells using MTT assays. Results from 24 h incubation tests indicate that the hydrochromic dyes we used here are within low toxicity range (see Supplementary Fig. 11 ). Toxicological tests over extended periods of exposure to the dyes with mice are in progress, and these results will be reported later as a continuation of this work. We need to point out that, as the dyes we used here are insoluble in water, the potential problem of dye exposure upon human contact is eliminated after a non-toxic PEG-capping layer is used for the RP material. The current rewritable prototype is easily compatible with commercially available ink-jet printers by simply replacing ink with water in the cartridges. This simple water-refilling solves the primary problem of frequent replacement of ink cartridges associated with ink-jet users. To demonstrate the feasibility of our developed RP for the practical applications, we printed an A4 size water-jet prints in comparison with HP ink-jet prints ( Fig. 7 ). The legibility and resolution of our current water-jet prints seem good enough for general reading purpose, and we are confident to improve further the colour intensity and evenness of our rewritable media. 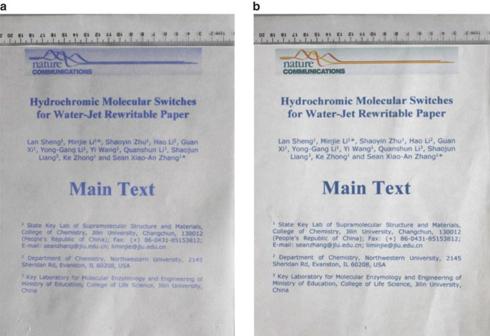Figure 7: Side-by-side comparison of water-jet prints with ink-jet prints. (a) Water-jet prints (210 × 297 mm) printed by HP DeskJet 2010 printer with cartridges (HP 704) refilled with water (4 ml) on ourRPbased on dye1. (b) Ink-jet prints (210 × 297 mm) printed by the same printer with commercial HP 704 black and tricolour cartridges. Figure 7: Side-by-side comparison of water-jet prints with ink-jet prints. ( a ) Water-jet prints (210 × 297 mm) printed by HP DeskJet 2010 printer with cartridges (HP 704) refilled with water (4 ml) on our RP based on dye 1 . ( b ) Ink-jet prints (210 × 297 mm) printed by the same printer with commercial HP 704 black and tricolour cartridges. Full size image According to a rough estimation, the cost per print of the RP (based on a conservative 10 times reusage/sheet) would be approximately one-seventeenth of the normal ink-jet print (see Supplementary Table 2 ). Even though the 22 h legible image-lasting time accomplished so far is not long enough for keeping records, this still provides a good alternative for reducing paper waste from temporary reading. Furthermore, our rewritable paper overcomes some disadvantages of the current version of rewritable media, including higher cost and more energy consumption. In summary, we present a green and economic strategy to develop ink-free rewritable paper by introducing hydrochromic dyes in paper and using water as the sole trigger. Important insights on the relationship of the molecular structures with their hydrorchromic properties have been obtained, which allow us to screen and identify quickly the ideal candidates to be used for the imaging materials. Negative impacts on the practical usage of the rewritable dyes from the fixed spatial polyhydroxyl environment of the paper, microcrystalline aggregation and excessive ambient moisture have been successfully overcome. A prototype of ink-free RP with legibility lasting nearly one full day per print under normal ambient conditions has been developed, and dozens of write–erase cycles without obvious colour fading have been realized. This water-jet rewritable printing is pointing a very good direction on green life, and will inspire further development of better rewritable media for global sustainable growth. Synthesis of compounds 1–10 General procedure I for synthesis of A1 – 10 : The phenylhydrazines (1 equivalent (eq. ), 3-methyl-2-butanones (1.3 eq.) and H 2 SO 4 (0.1 eq.) were dissolved in glacial acetic acid and then heated under reflux for 7.5 h under nitrogen. After the reaction was cooled to room temperature, the solvent was evaporated in vacuo . The residue was dissolved in CH 2 Cl 2 , washed with 10% aqueous Na 2 CO 3 and dried with anhydrous Na 2 SO 4 . Then CH 2 Cl 2 was removed in vacuo. The products were obtained using vacuum distillation or purified using column chromatography to afford A1 – 10 . General procedure II for synthesis of B1 – 10 : A1 – 10 (1 eq.) and 2-bromoethanol (1.2 eq.) were dissolved in MeCN and heated under reflux for 25 h under nitrogen, and then the reaction was allowed to cool to room temperature. The precipitate was filtered and washed with Et 2 O. The resulting solids were collected and recrystallized from EtOH/EtOAc to afford B1–10 . General procedure III for synthesis of C1 – 10 : B1 – 10 (1 eq.) and aromatic aldehydes ( D1–10 ) (1.2 eq.) were dissolved in EtOH under nitrogen with the addition of three drops of CH 3 SO 3 H as a catalyst. The solution was maintained at reflux for 6 h before stopping the heat. The reaction was then allowed to cool to room temperature. The resulting precipitate was washed by EtOAc to afford crude products. The crude products were recrystallized from EtOAc/hexane to afford C1 – 10 as solids. General procedure IV for synthesis of 1 – 10 : C1 – 10 were basified by adding 5% NaHCO 3 aqueous solution until the solution turned brown, at which point the solutions were extracted with EtOAc. The organic layers were collected, dried over anhydrous Na 2 SO 4 and concentrated to afford 1 – 10 as solids. Preparation of rewritable papers The rewritable paper integrated with 1 was prepared in a layer-by-layer manner. The filter paper substrate was coated with a layer of 10 wt% PEG aqueous solution and dried at 70 °C. Then EtOH/H 2 O (2/3 by volume) solution of 1 (0.08 mmol l −1 ) containing 6 wt% PEG and 0.01 wt% of NaNO 3 as the hydrating agent is coated over the initial PEG layer. Lastly, another protective layer of PEG was coated on the top using 10% PEG aqueous solution after the first two layers were dried completely. Layer-by-layer coating methods and procedures as these used for 1 were used for the fabrication of rewritable paper based on 2 , 3 and 4 . Owing to the different sensitivities of these molecules to the hydroxyl groups on the surface of the filter paper, the contents of each passivation layer varied slightly. The passivation layer for 2 was prepared from a 10% PEG aqueous solution with 1 mmol l −1 NaHCO 3 . The passivation layer for 3 was prepared from a 10% PEG aqueous solution. The passivation layer for 4 was prepared from a 20% PEG aqueous solution. PEG 20000 (molecular weight: 17,000–22,000) was purchased from GUANGFU fine chemical research institute (Tianjin, China). Cellulose filter paper (Whatman–Xinhua, grade 91, Hangzhou, China) is selected as the paper substrate. Cell cytotoxicity test condition HeLa cells (a human epithelial cervical cancer cell line) were cultivated at 37 °C under humidified 5% CO 2 in Dulbecco’s modified Eagle’s medium, supplemented with 10% fetal bovine serum and 100 μg ml −1 penicillin–streptomycin. HeLa cells were seeded in 96-well tissue culture plates at a density of 5,000 per well in Dulbecco’s modified Eagle’s medium containing 10% fetal bovine serum. The cytotoxicity of the dyes was evaluated by determining cell viability after 48 h of incubation with various final concentrations of 1–4 (0.3−30 μg of dyes ml −1 ). The number of viable cells was determined by estimating their mitochondrial reductase activity using the tetrazolium-based colorimetric method (MTT conversion test) with a Microplate Reader (GF-M3000, Caihong, China) at a wavelength of 495 nm. The relative cell viability (%) for the controls (containing cell culture medium) was calculated as: test/control × 100. How to cite this article: Sheng, L. et al . Hydrochromic molecular switches for water-jet rewritable paper. Nat. Commun. 5:3044 doi: 10.1038/ncomms4044 (2014).